Ravens notice dominance reversals among conspecifics within and outside their social group A core feature of social intelligence is the understanding of third-party relations, which has been experimentally demonstrated in primates. Whether other social animals also have this capacity, and whether they can use this capacity flexibly to, for example, also assess the relations of neighbouring conspecifics, remains unknown. Here we show that ravens react differently to playbacks of dominance interactions that either confirm or violate the current rank hierarchy of members in their own social group and of ravens in a neighbouring group. Therefore, ravens understand third-party relations and may deduce those not only via physical interactions but also by observation. The ‘social brain hypothesis’ (SBH) [1] , [2] , [3] attributes the evolution of intelligence to the cognitive demands of social life. In support of the SBH, measures of social complexity and/or competence are found to correlate with neocortex size [3] and reproductive success [4] , [5] , [6] . Furthermore, the type and quality of social relationships turns out to play a key role in several vertebrate societies, irrespective of group stability and the degree of fission–fusion dynamics [7] , [8] , [9] , [10] . Species living with long-term pair partners, for instance, tend to have bigger brains than those forming short-term or seasonal relations [11] , [12] . The exceptions are primates, possibly because their social life requires them to deal not only with one but several long-term relationships at a time [3] . Indeed, primates, not only recognize others as kin, friend or dominant but also understand third-party relationships within these kin-, friendship- and/or dominance networks [13] , [14] , [15] , [16] , [17] . A similar picture has been discussed for spotted hyenas, which live under social conditions comparable to primates [18] . Recently, the SBH has been extended to birds [19] and used to explain the apparent case of convergent evolution of intelligence in apes and corvids [20] . However, evidence that birds have an understanding of social dynamics similar to that of mammals is still scarce. For example, although several bird species seem to be capable of transitive inference [21] , [22] , [23] , [24] , [25] (but see ref. 26 ), only two species have been experimentally tested for using this capacity to predict their own dominance status compared with that of a stranger [27] , [28] . Note that these inferences are based on recent events, that is, seeing others winning or losing against a known individual, and do not necessary require knowledge about the relationship between the other individuals. The experiments clearly show, however, that the birds readily used the experience they had with one of the combatants from previous encounters. In the studies on primates and hyenas, the classification of relative rank relations also concerned group members they had ample interactions with in daily life [28] . It thus remains unknown whether non-human animals can deduce social relations such as relative rank between individuals they can observe but not interact with themselves. As the largest and most widely distributed member of the corvid family, ravens are renowned for their relatively big brains and high behavioural and ecological flexibility [29] . Their cognitive skills are expressed primarily in the social domain: on one hand, they flexibly switch between group foraging (including active recruitment) [30] and individual strategies (like providing no or false information about food, attributing perception and knowledge states about food caches to others) [31] ; on the other hand, they form and maintain affiliate social relations aside from reproduction and engage in primate-like social strategies like support during conflicts [32] , and reconciliation and consolation after conflicts [33] . Understanding social relations of others may be key in those behaviours. Ravens also remember former group members and their relationship valence over years [34] , which might be important for life in non-breeder flocks where some individuals stay together over extended periods of time, whereas others do not [35] . A consequence of these dynamics is that ravens regularly meet conspecifics of different degrees of familiarity, many of which they have never interacted with before. As dominance rank heavily depends on affiliation status and social support by others [35] , raven non-breeders are ideal to test for the ability of third-party understanding between birds that regularly interact but also of those that know each other merely by observation. Therefore, here we tested 16 captive common ravens, Corvus corax , on their ability to recognize third-party rank relations of individuals they regularly interact with (group members) and those they do not (neighbouring group) by use of a playback experiment applying an expectancy violation paradigm [5] . In this study we show that ravens react differently to playbacks of expected and unexpected dominance interactions of conspecifics. Consequently, ravens seem to understand third-party rank relations. As they do so, both of individuals within their own group as well as of individuals in a neighbouring group, we suggest that ravens are capable of forming representations of others’ relationships that are entirely based on observation of other’s interactions. Playbacks of group members The final generalized linear mixed models (GLMM’s) on the delta-scores of in-group playbacks showed that ravens became more stressed and showed more self-directed behaviour when the playback violated their expectancy of rank relations compared with playbacks of expected interaction, since the models revealed a significant effect of treatment (expected versus unexpected) on self-directed behaviour (GLMM: F =7.09, df 1 =1, df 2 =57, P =0.010; Fig. 1a ) and a similar, yet non-significant trend for ‘stress’ behaviour (GLMM: F =3.93, df 1 =1, df 2 =57, P =0.052; Fig. 1b ). 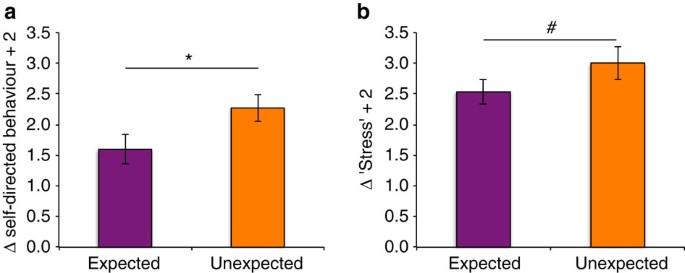Figure 1: Self-directed and ‘stress’ behaviour in response to in-group stimuli. Mean±s.e.m. difference between playback and baseline (delta:Δ) of (a) self-directed behaviour and (b) ‘Stress’ behaviour, for playbacks simulating expected (purple bars) and unexpected (orange bars) dominance interactions of in-group individuals. For clarity, we added 2 to these means.n=16, GLMM: *P<0.05,#0.05<P<0.10. Figure 1: Self-directed and ‘stress’ behaviour in response to in-group stimuli. Mean±s.e.m. difference between playback and baseline (delta: Δ ) of ( a ) self-directed behaviour and ( b ) ‘Stress’ behaviour, for playbacks simulating expected (purple bars) and unexpected (orange bars) dominance interactions of in-group individuals. For clarity, we added 2 to these means. n =16, GLMM: * P <0.05, # 0.05< P< 0.10. Full size image In addition, the models showed an interaction effect between the sex of the subject and condition on self-directed behaviour (GLMM: interaction sex × condition: F =5.49, df 1 =1, df 2 =57, P =0.023; Fig. 2 ), suggesting that the main effect of condition is mainly due to the females. Post hoc analyses indeed revealed that females reacted with significantly more self-directed behaviour after an unexpected playback compared with an expected playback (Wilcoxon-signed ranks test: T + =44, n =9, P =0.011), whereas for males this difference was non-significant ( Fig. 2 ). Furthermore, the models showed that compared to baseline, individuals became more active when their expectancy was violated, yet only when it concerned playbacks of their own sex (GLMM: interaction sex−combination × condition: F =6.65, df 1 =1, df 2 =57, P =0.013; Fig. 3 ). Post hoc analyses confirmed that individuals became significantly more active when they heard an unexpected playback compared with an expected playback of their own sex (Wilcoxon-signed ranks test: T + =123, n =16, P =0.004), whereas this difference was non-significant when the playback concerned individuals of the other sex ( Fig. 3 ). Finally, we found significant effects of age on the components activity (GLMM: F =9.401, df 1 =1, df 2 =57, P =0.003), attention (GLMM: F =4.34, df 1 =1, df 2 =57, P =0.042) and ‘stress’ (GLMM: F =4.71, df 1 =1, df 2 =57, P =0.034), indicating that compared to baseline, older individuals reacted with more activity, less interest and more stress to playbacks in general, regardless of their congruence ( Supplementary Fig. 1 ). 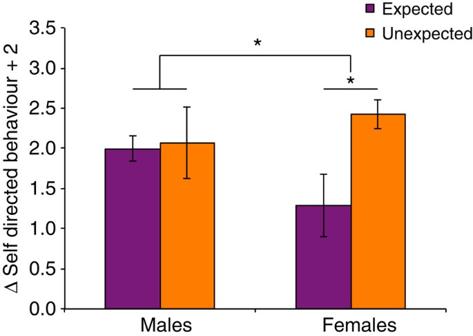Figure 2: Sex differences in self-directed behaviour in response to in-group stimuli. Mean±s.e.m. difference between playback and baseline (Δ) self-directed behaviour of males (n=7) and females (n=9), for playbacks simulating expected (purple bars) and unexpected (orange bars) dominance interactions of in-group individuals. For clarity, we added 2 to these means. GLMM andpost hocWilcoxon-signed ranks tests: *P<0.05. Figure 2: Sex differences in self-directed behaviour in response to in-group stimuli. Mean±s.e.m. difference between playback and baseline ( Δ ) self-directed behaviour of males ( n =7) and females ( n= 9), for playbacks simulating expected (purple bars) and unexpected (orange bars) dominance interactions of in-group individuals. For clarity, we added 2 to these means. GLMM and post hoc Wilcoxon-signed ranks tests: * P <0.05. 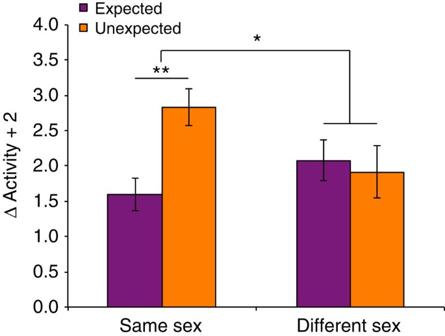Figure 3: Activity in response to in-group stimuli of the same or of the other sex. Mean±s.e.m. difference between playback and baseline (Δ) of activity, for playbacks simulating expected (purple bars) and unexpected (orange bars) dominance interactions of in-group individuals of the same sex and of individuals of the different sex. For clarity, we added 2 to these means.n=16, GLMM andpost hocWilcoxon-signed ranks tests: *P<0.05; **P<0.01. Full size image Figure 3: Activity in response to in-group stimuli of the same or of the other sex. Mean±s.e.m. difference between playback and baseline ( Δ ) of activity, for playbacks simulating expected (purple bars) and unexpected (orange bars) dominance interactions of in-group individuals of the same sex and of individuals of the different sex. For clarity, we added 2 to these means. n =16, GLMM and post hoc Wilcoxon-signed ranks tests: * P <0.05; ** P <0.01. Full size image Playbacks of neighbouring group Regarding the playbacks of out-group conspecifics, we found no main effect of treatment on the behaviour of the ravens. However, we did find significant interaction effects of the sex of the subject with treatment on vocalization (GLMM: interaction sex−combination × condition: F =4.28, df 1 =1, df 2 =57, P =0.043) and on attention: (GLMM: interaction sex−combination × condition: F =4.05, df 1 =1, df 2 =57, P =0.049), suggesting that only males respond to violations of rank relations of out-group conspecifics. Compared with baseline, males reduced their vocalizations when the playback violated their expectancy of rank relations significantly more than during playbacks of expected interaction (Wilcoxon-signed ranks test: T + =26, n =7, P =0.043), whereas for females this difference was non-significant ( Fig. 4a ). Similarly, males tended to reduce their behaviours indicative of showing attention compared with baseline more when the playback was unexpected than when it was expected (Wilcoxon-signed ranks test: T + =24, n =7, P =0.091), whereas for females there was no such trend ( Fig. 4b ). Finally, we found significant effects of the sex of the playbacked individuals on attention (GLMM: F =10.84, df 1 =1, df 2 =57, P =0.002) and self-directed behaviour (GLMM: F =5.23, df 1 =1, df 2 =57, P =0.026), suggesting that compared to baseline, individuals reacted with more interest, and less stress release to playbacks of same sex individuals in general, regardless of their congruence ( Supplementary Fig. 2 ). 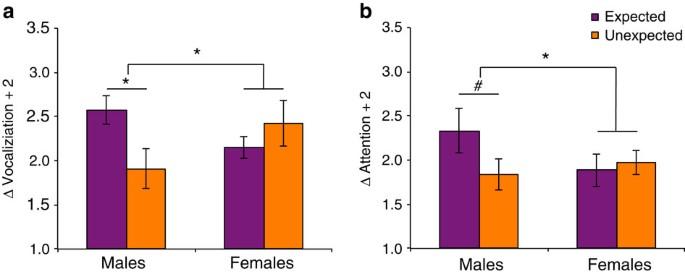Figure 4: Vocalizations and close interest behaviour of males and females in response to out-group stimuli. Mean±s.e.m. difference between playback and baseline (Δ) of (a) vocalizations and (b) close interest behaviour of males (n=7) and females (n=9), for playbacks simulating expected (purple bars) and unexpected (orange bars) dominance interactions of in-group individuals. For clarity, we added 2 to these means. GLMM andpost hocWilcoxon-signed ranks tests: *P<0.05,#0.05<P<0.10. Figure 4: Vocalizations and close interest behaviour of males and females in response to out-group stimuli. Mean±s.e.m. difference between playback and baseline ( Δ ) of ( a ) vocalizations and ( b ) close interest behaviour of males ( n =7) and females ( n =9), for playbacks simulating expected (purple bars) and unexpected (orange bars) dominance interactions of in-group individuals. For clarity, we added 2 to these means. GLMM and post hoc Wilcoxon-signed ranks tests: * P <0.05, # 0.05< P< 0.10. Full size image Our results reveal that ravens show different behaviour after playbacks that simulate a rank reversal in their group in comparison with playbacks that suggest dominance interactions in line with the current dominance hierarchy. These findings demonstrate that ravens, just like primates [13] , [14] , [15] , [16] , [17] , can distinguish these different types of playbacks and thus have some knowledge about the rank relations of their group members. Furthermore, male ravens responded to playbacks violating the dominance relations of their neighbouring group. This is, to our knowledge, the first experimental demonstration that non-human animals may recognize the rank relations of out-group members. Moreover, these findings strongly suggest that ravens are capable of forming representations of others’ relationships that are entirely based on observation of other’s interactions. Owing to our controlled captive set-up, we can exclude that subjects had any experience of physically interacting with members of the neighbouring group before testing. Hence, the subjects’ own ranks were independent of the ranks of the out-group members being played back, and the rank relations of out-group members could not be deduced through comparison of the absolute rank differences between the played back individuals and the tested individual (that is, the focal subject’s own rank relative to those of others). A prevailing criticism on similar playback experiments in primates is that individuals just react more strongly to distress/submissive calls from more dominant individuals as these occur less frequently. However, out of 12 individuals used to combine the stimuli, we only included one top-ranking bird that only recently before the study became the dominant male in its group. Moreover, the ranks of the individuals that produced the submissive call in our playbacks could not significantly predict any of the response variables in both the in- and the out-group condition, respectively (GLMM: P >0.05). Thus, the effect cannot be explained by simple habituation to the submissive calls of lower-ranking birds. Furthermore, the different response patterns to in- and out-group members indicate that the played back stimuli were meaningful to the birds. All ravens tended to react with an increase in ‘stress’ behaviour, and particularly females reacted with an increase in self-directed behaviours, which often correlates with the reduction of stress [36] , [37] , to simulated rank reversals in their own group. Furthermore, all ravens increased activity levels when the simulated rank reversal was about members of their own sex, that is, when it concerned the position close to their own in the rank hierarchy. Consequently, (simulated) rank reversals in their own group seem stressful for ravens, especially when these reversals happen in positions close to your own rank (same sex) or when you are low in the dominance rank hierarchy (females [35] , [38] ). In contrast, when the playback concerned simulated rank reversals in the neighbouring group, they showed no signs of stress or activity but a change in vocalization and attention. Interestingly, they decreased these behaviours during violations, suggesting that they were prone to display interest to simulated interactions of known rather than unknown outcome. This corresponds to the observations that ravens are excellent in monitoring, and actively intervening, in status-related interactions of other ravens [34] and the findings of previous playback experiments that ravens show a stronger vocal response to familiar than to unfamiliar conspecifics [34] . A sophisticated use of bystander information has also been found in the context of food caching, including judging the others’ perspectives and possibly even knowledge sates [31] . Aside studies on transitive inference [21] , [22] , [23] , [24] , [25] , [27] , [28] , the current study provides the first experimental test for third-party knowledge in birds that is based on an expectancy violation paradigm as used in mammals [5] ; yet our results fit well to the selectivity in third-party interventions of corvids observed under daily life conditions [12] , [32] and to the increase in heart rate measured in bystanders of third-party interactions in free-ranging graylag geese [39] . Taken together, these findings support the hypothesis that understanding the relationships between others is critical for navigating in a complex social world not only in mammals but also in birds. Interestingly, the social life of most birds with its relatively high degree of fission–fusion dynamics over seasons and years [35] is quite different from that of the well-studied primates like baboons and vervet monkeys, which live in relatively stable groups [40] . Yet, social bonds and pairbond-like friendships are highly important in corvids and the other avian species of interest [11] , [12] , creating a system of dependent ranks. This is especially true for female ravens, which substantially gain in rank by bonding to males [35] . The crucial role of males in raven society for gaining and maintaining status might be the reason why only males responded to simulated rank reversals in the out-group condition of our experiment. Future studies may show whether females do not know about these relations or just did not show a response in this set-up. On the basis of the current results, we argue that both male and female ravens understand the third-party rank relations of those individuals they regularly interact with (their own group), and that by mere observation male ravens also seem to have a representation of the rank relations of the members of a neighbouring group. Subjects and housing We used 16 sub-adult captive ravens housed in two separate social groups of eight birds each at the Haidlhof Research Station, Bad Vöslau, Austria. Both groups contained male and female peers (group 1: 3 males, 5 females; group 2: 4 males, 4 females). For a description of each individual (for example, age, rank and raising history) see Supplementary Table 1 . Both groups were kept in adjacent parts of a large aviary complex (compartment A and B; Fig. 5a ) for 9 months, with full visual and auditory access to the other group. Before the experiments, during a 1-month period, each group was trained to temporarily use another part of the complex, that is, birds of group 1, that traditionally were found in part B, could move to part C; birds of group 2, that traditionally used part A, could move to part B when group 1 was in C ( Fig. 5b ). This procedure allowed us to familiarize birds of both groups with the middle compartment B, which was subsequently used for testing. All aviary parts are enriched with trees, perches, playing devices and shallow pools for bathing. The middle compartment B is subdivided into two same-sized parts (B-I, B-II) by wire mesh panels with sliding doors and an opaque observation hut (2.5 × 2.5 m 2 ). On experimental days, the birds received their normal diet consisting of meat, milk products, bread, vegetables and fruits twice a day. Water was available ad libitum . 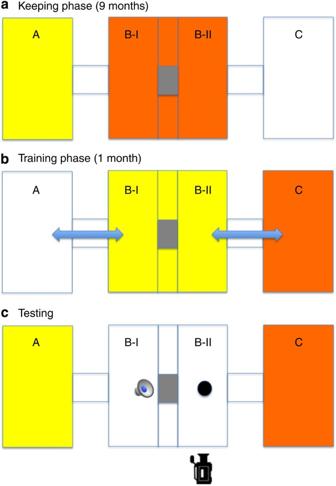Figure 5: Schematic representation of the set-up of the aviaries. Aviaries A (18 × 10 × 5 m3), B (15 × 15 × 5 m3) and C (8 × 10 × 5 m3), housing group 1 (orange) and group 2 (yellow) during the different phases (a–c) of the experiment. The black dot represents an example of an animal in a test, the sound logo the place of the speaker from which the playback was played and the camera logo the respective place of the cameras that filmed this bird. Figure 5: Schematic representation of the set-up of the aviaries. Aviaries A (18 × 10 × 5 m 3 ), B (15 × 15 × 5 m 3 ) and C (8 × 10 × 5 m 3 ), housing group 1 (orange) and group 2 (yellow) during the different phases ( a – c ) of the experiment. The black dot represents an example of an animal in a test, the sound logo the place of the speaker from which the playback was played and the camera logo the respective place of the cameras that filmed this bird. Full size image Ethical note The ravens of group 1 originated from captive breeding pairs in zoos (Alpenzoo Innsbruck, Austria; Zoo Wels, Austria; and Nationalpark Bayrischer Wald, Germany) and a private owner (K Trella, Austria); those of group 2 originated from captive breeding pairs at the Konrad Lorenz Forschungsstelle in Grünau, Austria and from Lund University, Sweden. The study complied with Austrian law and local government guidelines (§ 2. Federal Law Gazette number 501/1989), and received oversight from the internal behavioural research group at the faculty of Life sciences, University of Vienna, and was authorized owing to its non-invasive character. The study subjects remained in captivity at Haidlhof Research Station after the completion of this study for further research. Experimental design and set-up Experiments started after all birds were comfortable with a short individual separation in the middle compartment B, while their conspecifics remained in parts A and C. For testing, the focal subject was called either into subdivision B-I or B-II, that is, in the half being closer to A or C, respectively; the loudspeaker used for playing back the stimuli was hidden in the opposite subdivision, always behind the wooden hut. Specifically, the loudspeakers’ position was such that the direction of the played back stimuli was congruent with the current position of the group that particular stimuli could come from: if the focal subject was positioned in B-I, it was tested with stimuli of group 1 from the direction of C; if it was positioned in B-II, it was tested with stimuli of group 2 from the direction of A ( Fig. 5c ). Each playback contained three vocal interactions of the same individuals, each separated by 1 min. Stimuli were played from a loudspeaker (LD systems Roadboy 65, flat frequency response 80–15 kHz) connected to a MacBook Pro through a wireless system (Sennheiser EK 2000, flat frequency response 25–20 kHz). Loudness was adjusted to the natural submissive vocalization sound pressure levels. The actual playback loudness at the receiver varied depending on focal bird’s position in the aviary and the weather conditions. To hinder social learning and/or disruption of established hierarchies, the test playbacks were masked for all other animals using synchronized white-noise playbacks from two loudspeakers (LD systems Roadboy 65, flat frequency response 80–15 kHz), one directed at each groups. All loudspeakers were visually occluded for all animals. Conditions Focal individuals were subjected to playbacks of vocal interactions (see acoustic information below) of two other birds in an order consistent with the group’s dominance hierarchy (expected condition) and in an order inconsistent (that is, mimicking a rank reversal) with the group’s dominance hierarchy (unexpected condition). Per testing day, the birds received two sessions: one with playbacks of individuals of their own sex and one with playbacks of individuals of the different sex. In addition, animals were tested twice: once with playbacks of group members (both males and females) and once with playbacks of members of the other group (again both males and females). Consequently, all birds were tested in four conditions per in/out-group; that is, two control (expected) and two corresponding test (unexpected) conditions. The order of expected versus unexpected was counterbalanced over the tested birds within each session, the order of the played back sexes was counterbalanced over the tested birds over the two sessions per day and the order of in- or out-group playbacks were counterbalanced over the tested birds over the two testing days. For a schematic representation of all conditions please see Supplementary Table 2 . Testing lasted roughly an hour per day: after a 15-min habituation period, we played back the first stimulus to the subject (session 1, for example, own sex/congruent), and after another 15 min, we played back the second stimuli (session 2, for example, own sex/incongruent), followed by 15 min post observations. For the entire period, the behaviour of the focal subject was videotaped (using two Canon LEGRIA HD-camcorders). Models (that is, those individuals whose calls were played back) remained the same per focal subject, that is, both the expected and unexpected playback of either familiar (in-group) or unfamiliar (out-group) and of either same-sexed and different-sexed birds. For an overview of which models were used for which subject, please see Supplementary Table 1 . Acoustic recordings and stimuli preparation The playback consisted of two types of vocalizations: self-aggrandizing display (hereafter SAD) and submissive calls [41] . Ravens of both sexes show SADs accompanied by a dominant posture, as a directed dominance display, which is often followed by submissive calls ( Supplementary Fig. 3 ), and submissive posture and retreat by the subordinate individual. Note that the combination of SADs and submissive calls determined the meaning of the interaction, that is, a mild conflict with clear outcome. Ravens can show SADs also in a non-directional way, typically when they have temporarily left or are about to join the group. Acoustically, SADs can be highly variable between regions and individuals [41] and a single individual may produce several distinct SAD types (personal observation). In our case, most birds within each group shared their vocal display repertoire regardless of their sex but varied in the frequency of certain SAD type usage ( Supplementary Fig. 4 ). To create the stimuli, we used the two predominant SAD types from each group ( Supplementary Table 3 ). We constructed the dyadic interaction stimuli using vocalizations of six birds (three males and three females of consecutive ranks) from each group. Each stimulus approximated a dyadic interaction of a dominant (SAD vocalization) and subordinate (submissive vocalization) individual. We used the most frequent SAD type for each bird ( Supplementary Table 3 ). Only within-sex interactions were considered. For each sex and group, this resulted in four stimuli of one rank step (two congruent and two incongruent with the actual group hierarchy) and two stimuli of two rank steps. In total, we obtained 24 playback stimuli (two groups × two sexes × three individuals × two congruency conditions). Acoustic recordings of SADs and submissive calls were obtained between February 2011 and June 2012 from various non-experimental situations. All calls were recorded with a Sennheiser K6/ME66 shotgun microphone connected to a Marantz PMD660/Zoom H4n digital recorder or a Canon LEGRIA HD-camcorder. Best quality recordings were individually extracted, high-pass filtered at 200 Hz and peak amplitude normalized. SADs were normalized at −10 dB levels of the submissive calls to approximate the natural loudness difference between the two call types. Submissive calls are usually produced in bouts, which include adjacent calls without pause. For better approximation of the natural call occurrence, submissive calls were extracted singly or as two immediately adjacent calls. Each individual stimulus consisted of a bout of three SADs from individual I immediately followed by a bout of five to seven submissive calls from individual II followed again by a single SAD from individual II ( Fig. 6 and Supplementary Audio 1 ). SADs were spaced 2±0.2 s and submissive calls <0.5 s apart. The number of submissive calls varied between five and seven depending on the length of the individual calls in the stimulus. All individual calls were used no more than once within one stimulus and no more than three times within one playback session. We prepared stimuli using PRAAT 5.2.46 (ref. 42 ) and Adobe Audition CS5.5 software packages for mac OS X. 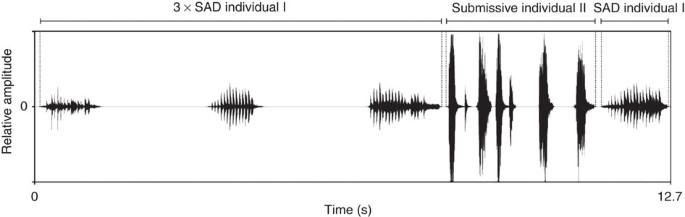Figure 6: Example waveform of a playback stimulus. Playback stimulus simulating an interaction between a dominant bird giving a bout of three SADs (individual I) followed by a bout of submissive vocalizations from a subordinate bird (individual II) and followed again by one SAD from the dominant. Figure 6: Example waveform of a playback stimulus. Playback stimulus simulating an interaction between a dominant bird giving a bout of three SADs (individual I) followed by a bout of submissive vocalizations from a subordinate bird (individual II) and followed again by one SAD from the dominant. Full size image Measures and data analyses Before the experiments, we analysed the dominance hierarchies in both groups. Therefore, we provided the birds with a heap of food that could be monopolized by one individual and scored all unidirectional displacements [38] . We arranged these data in matrices with actors in rows and recipients in columns. We determined the dominance order most consistent with a linear hierarchy, calculating Landau’s linearity indices ( h ′) using MatMan 1.1 (ref. 43 ) and reordered matrices to best fit a linear hierarchy [44] , [45] . We found significantly linear hierarchies in both groups (group 1: h′ =0.964, n =8, P <0.001, based on 342 interactions and with 0% unknown relationships; group 2: h′ =0.774, n =8, P =0.015, based on 403 interactions and 3.57% unknown relationships). Videos of the experiments were coded with Solomon coder [46] by J.S. who was blind for the congruence of the playback and for the sex of the played back individuals. Per playback, we coded 17 different behavioural variables (see Supplementary Table 4 ) during the 3.5 min of the playback (three playbacks a 10 s+2 min in between the three playbacks and 1 min post playback) and during the 3.5 min before the playback. Playbacks (12.5%) were recoded by Kerstin Pölzl. We used Spearman’s ρ -correlations to calculate inter-rater reliability regarding durational behaviours. All durational measures were scored almost identically, with Spearman’s ρ -correlation coefficients ranging between 0.73 and 1, and P ≤0.001. Inter-rater reliability regarding point behaviours was calculated using Cohen’s κ . The value of κ was 0.68, which corresponds to a good level of agreement (91.2% agreement). To reduce the amount of response variables, we performed a principle component analysis (PCA) on all behaviours coded during and before the playback. Note that if different sets of behaviours are found together before and after the playback, combining the two times might be hindering the PCA. Subtracting the behaviours found during the playback from the baseline before playback may lessen this problem. However, such a subtraction presumes an a priori difference between the phases, which would cause a problem for a subsequent PCA in case this difference is not present owing to a large amount of zeros in the data. On the basis of eigenvalue (>1) and scree-plot investigation, we extracted five components that in total explained 53.4% of the overall variance of all data. On the basis of the variable loadings, the five components seem to reflect; 1, activity; 2, vocalization; 3, attention; 4, self-directed behaviour; and 5, ‘stress’ ( Supplementary Table 4 ). Subsequently, we procured individual component scores for the five PCA components using the regression method. These component scores have a mean of zero and a variance equal to the squared multiple correlation between the estimated and the true component values. To assess whether individuals reacted differently to playbacks with an expected interaction versus a playback with an unexpected interaction, we first calculated per component the difference between an individual’s component score during and before the playback that is, playback−baseline (delta). Per component, we then used GLMM to assess the effect of condition (expected versus unexpected), sex of the subject, sex of the playback and age on the delta score. We ran separate analyses for the responses to in-group and to out-group stimuli. In these models, the delta of the component scores was the response variable, whereas condition, sex, sex of the playback and age were entered as fixed variables. Furthermore, as we dealt with repeated data, we structured our data as to represent the nested structure of our data. Particularly, we structured our data to be nested in each individual, which in turn were nested in one of the two groups. Consequently, we entered subject identity and group as random variables to our models. We ran models including all main effects and two-way interactions of sex and sex of the playback with condition, and several reduced models and selected the best fitting model with the Akaike Information Criteria. All reported P -values are two tailed, and we consider α ≤0.05 as a significant effect. Where appropriate, we ran post hoc analyses using Wilcoxon-signed ranks tests. How to cite this article: Massen, J. J. M. et al. Ravens notice dominance reversals among conspecifics within and outside their social group. Nat. Commun. 5:3679 doi: 10.1038/ncomms4679 (2014).